O-glycosylation modulates integrin and FGF signalling by influencing the secretion of basement membrane components Extracellular microenvironments have crucial roles in modulating cell interactions during development. Here we discover that a conserved protein modification (O-glycosylation) influences extracellular matrix composition during mammalian organogenesis, affecting integrin signalling and fibroblast growth factor-mediated cell proliferation. Specifically, mice deficient for an enzyme ( Galnt1 ) that adds sugars to proteins during early stages of organogenesis resulted in intracellular accumulation of major basement membrane proteins and endoplasmic reticulum stress, with resultant effects on fibroblast growth factor signalling, epithelial cell proliferation and organ growth. Exogenous addition of basement membrane components rescued fibroblast growth factor signalling and the growth defects in a β1-integrin-dependent manner. Our work demonstrates for the first time that O-glycosylation influences the composition of the extracellular matrix during mammalian organ development, influencing specific aspects of the endoplasmic reticulum stress response, cell signalling, cell proliferation and organ growth. Our work provides insight into the role of this conserved protein modification in both development and disease. The cellular microenvironment is a vast array of components that surround cells and tissues, modulating basic processes such as cell adhesion, differentiation, proliferation and signalling. The crucial importance of this extracellular matrix (ECM) is illustrated in diseases where changes in the constitution of the matrix are accompanied by altered cell proliferation and morphology, associated with tumour progression and metastasis [1] , [2] , [3] , [4] . Although many factors are known to influence the composition of the cellular environment, the inherent complexities associated with the synthesis, processing, transport and secretion of the diverse components indicate many levels of regulation that are yet to be discovered. The basement membrane (BM) is a specialized ECM microenvironment surrounding all epithelia during mammalian development. BMs form structural scaffolds for tissue morphogenesis, and also regulate cell proliferation and signalling events during development by serving as ligands for receptors as well as reservoirs for growth factors and other bioactive molecules [5] , [6] . The two major BM components present in developing mammalian organs are collagen and laminin. While collagen mediates BM stability in many developing tissues, laminin is required for BM formation, as mice deficient in laminin α1, β1 or γ1 lack BMs and die during early embryogenesis [5] , [6] . Murine embryonic submandibular gland (SMG) development and growth are regulated by components of the BM [7] , [8] , [9] , [10] , [11] , [12] . Intact collagen IV present within the BM provides structural integrity [5] , while the proteolytic NC1 fragments serve to regulate epithelial proliferation and end-bud expansion via PI3K-AKT signalling [11] . Likewise, laminin within the BM serves as both a scaffold for cell-matrix interactions as well as a ligand that mediates fibroblast growth factor (FGF) signalling through β1 integrin receptors [6] , [12] . Roles for the ECM proteins perlecan and fibronectin in gland clefting and growth have also been demonstrated [7] , [10] . Components of the BM are also rich in sugar-based modifications, including heparan sulfate glycosaminoglycans and O-linked glycans [10] , [13] , [14] . Specific glycosaminoglycans structures modulate FGF signalling by influencing receptor-ligand interactions [10] , [14] . However, the roles for additional sugars present within the BM are unknown. Recent work highlights the critical regulatory roles of sugar-based protein modifications in many aspects of development and disease [15] , [16] , [17] , [18] , [19] , [20] , [21] . The two major types of sugar linkages present on secreted proteins are N-linked (to asparagine) and O-linked GalNAc (to serine or threonine). N-linked glycosylation regulates protein folding, secretion and stability; disruption of N-glycosylation activates all branches of the endoplasmic reticulum (ER) stress response and induces cellular apoptosis [22] , [23] . Roles for O-linked glycosylation have been more difficult to decipher given the functional redundancy present among the 20 enzymes (ppGalNAcTs) responsible for initiation of this type of glycosylation in mammals [16] , [24] . While studies in model organisms have demonstrated that certain members of this family are essential for viability [25] , [26] , [27] , [28] , the redundancy present in mammals has hampered our understanding of the specific functions of these enzymes in human health and development. Nonetheless, alterations in protein O-glycosylation are associated with an increased risk of certain forms of cancer in humans, and are also responsible for two other diseases, familial tumoral calcinosis and Tn syndrome [29] , [30] , [31] , [32] , [33] . Additionally, genome-wide association studies have identified genes encoding O-glycosyltransferases among those associated with triglyceride and high-density lipoprotein cholesterol levels, thus implicating protein O-glycosylation in cardiovascular disease risk [34] , [35] , [36] . Although these studies highlight the impact of this evolutionarily conserved modification in human health, the mechanistic basis for the specific role of O-glycosylation in mammalian development and disease is largely unknown. Here we investigate the function of protein O-glycosylation during mammalian organogenesis by examining mice deficient for the O-glycosyltransferase ppGalNAcT-1 (ref. 37 ). Loss of the gene encoding ppGalNAcT-1 ( Galnt1 ) reduces cell proliferation and SMG growth by specifically disrupting the secretion of BM components, resulting in decreased integrin and FGF signalling. Additionally, we provide evidence that loss of O-glycosylation induces a subset of ER stress responses that are distinct from those induced upon the loss of N-linked glycosylation. We propose that Galnt1 -dependent O-glycosylation specifically regulates the composition of the cellular microenvironment during development by influencing BM protein secretion. This work provides a mechanism by which the loss of O-glycosylation may contribute to disease susceptibility by influencing ECM composition and the proteostasis network. Loss of Galnt1 affects SMG growth during early development We used qPCR to determine which of the 19 murine Galnt gene family members were expressed during SMG development ( Supplementary Fig. S1a ). Galnt1 was found to be the most abundantly expressed family member in embryonic day 12 (E12) SMGs ( Supplementary Fig. S1b ), suggesting a potential role for Galnt1 during early stages of SMG development. SMG development begins at E11.5 and then at E12, the SMG is visible as an initial, single epithelial end bud on a duct, surrounded by condensing mesenchyme ( Fig. 1b ). As development proceeds, the end bud enlarges via epithelial cell proliferation and undergoes cleft formation to begin the process of branching morphogenesis. Successive rounds of proliferation and clefting, as well as duct specification and elongation, result in an arborized glandular structure at later stages of development. 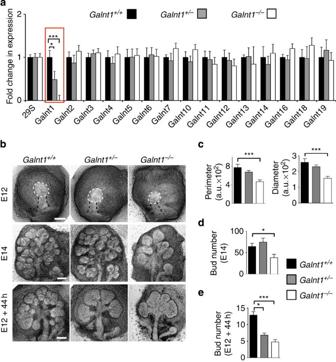Figure 1: Loss ofGalnt1results in smaller epithelial buds and reduced SMG growth. (a) Loss ofGalnt1expression (highlighted in red box) in SMGs fromGalnt1-deficient mice was verified by qPCR. Expression of otherGalntfamily members is unchanged inGalnt1-deficient SMGs. Expression was normalized to29S. (b) Loss ofGalnt1results in smaller E12 epithelial buds and reduced SMG growth. E12 SMGs from wild-type (Galnt1+/+;n=31),Galnt1heterozygotes (Galnt+/−;n=74) andGalnt1-deficient (Galnt1−/−;n=36) embryos were isolated and epithelial bud size (white dashed line) was measured. E14 SMGs fromGalnt1+/+(n=26),Galnt1+/−(n=38) andGalnt1−/−(n=16) were isolated and bud number was counted. E12 SMGs fromGalnt1+/+(n=9),Galnt1+/−(n=21) andGalnt1−/−(n=10) were grown for 44 h inex vivoculture and total bud number was counted. (c) Average perimeter and diameter of E12 epithelial buds from each genotype. (d) Average bud number present in E14 SMGs from each genotype. (e) Average bud number present after culturing each genotype for 44 h. Student'st-test was used to calculateP-values. *P<0.05; ***P<0.001. Figure 1: Loss of Galnt1 results in smaller epithelial buds and reduced SMG growth. ( a ) Loss of Galnt1 expression (highlighted in red box) in SMGs from Galnt1- deficient mice was verified by qPCR. Expression of other Galnt family members is unchanged in Galnt1- deficient SMGs. Expression was normalized to 29S . ( b ) Loss of Galnt1 results in smaller E12 epithelial buds and reduced SMG growth. E12 SMGs from wild-type ( Galnt1 +/+ ; n =31), Galnt1 heterozygotes ( Galnt +/− ; n =74) and Galnt1- deficient ( Galnt1 −/− ; n =36) embryos were isolated and epithelial bud size (white dashed line) was measured. E14 SMGs from Galnt1 +/+ ( n =26), Galnt1 +/− ( n =38) and Galnt1 −/− ( n =16) were isolated and bud number was counted. E12 SMGs from Galnt1 +/+ ( n =9), Galnt1 +/− ( n =21) and Galnt1 −/− ( n =10) were grown for 44 h in ex vivo culture and total bud number was counted. ( c ) Average perimeter and diameter of E12 epithelial buds from each genotype. ( d ) Average bud number present in E14 SMGs from each genotype. ( e ) Average bud number present after culturing each genotype for 44 h. Student's t -test was used to calculate P -values. * P <0.05; *** P <0.001. Full size image Galnt1 -deficient mice have been described previously as being viable but having lymphocyte homing defects and bleeding disorders of unknown etiology [37] . We examined the effects of Galnt1 loss on SMG growth and development by crossing Galnt1 +/− heterozygotes and analysing SMGs from wild type ( Galnt1 +/+ ), heterozygous ( Galnt1 +/− ) and Galnt1 -deficient ( Galnt1 −/− ) E12 littermates. qPCR analysis of SMGs demonstrated a specific loss of Galnt1 and no compensatory up or down regulation of other members of the family in Galnt1- deficient SMGs ( Fig. 1a ). E12 SMG buds from Galnt1 −/− animals were significantly smaller than both wild type and heterozygous littermates, as determined by measurement of the end-bud perimeter and diameter ( Fig. 1b,c ). Additionally, E14 SMGs from Galnt1 −/− animals were significantly smaller than littermate controls, as determined by counting the number of epithelial end buds ( Fig. 1b,d ). To determine whether the size differences observed between wild type and Galnt1 −/− E12 SMGs were due to an overall developmental delay in the Galnt1 −/− animals, we also examined E12 kidneys, another branching organ that expresses Galnt1 and develops at a similar time; however, Galnt1 is not the most abundant Galnt family member in this tissue. There were no significant size differences between the developing E12 kidneys from Galnt1 +/+ , Galnt1 +/− and Galnt1 −/− littermates ( Supplementary Fig. S2 ), suggesting that the differences observed are specific to the SMGs (where Galnt1 is the most abundant isoform) ( Supplementary Fig. S1b ). Examination of SMGs at later stages of development revealed that SMGs from Galnt1 −/− animals remain smaller into adulthood than Galnt1 +/+ littermate controls ( Supplementary Fig. S3 ). Ex vivo SMG organ culture was employed to examine the growth of Galnt1- deficient SMGs by quantifying the number of end buds present after culture. Interestingly, E12 Galnt1 −/− SMGs grew significantly slower than wild-type littermates in culture ( Fig. 1b,e ). Additionally, a less dramatic but significant reduction in growth was also seen for heterozygous Galnt1 +/− E12 SMGs grown in culture ( Fig. 1b,e ). Taken together, these results indicate that the loss of Galnt1 leads to reduced initial epithelial bud size and reduced SMG growth at early stages of development. Galnt1 -deficient SMGs have an altered BM composition It is known from previous studies that O-linked glycoproteins are typically abundant within the BM region of developing SMGs [13] . We therefore examined whether the epithelial BM was affected in Galnt1- deficient SMGs by staining for the major BM proteins (laminin and collagen IV) and total O-glycosylated proteins (as detected by the lectin peanut agglutinin, PNA) ( Fig. 2 ). Significant decreases in both laminin and collagen IV were seen within the BM of Galnt1 −/− SMGs when compared with wild type ( Fig. 2a,c,d ). Additionally, reductions in total O-glycosylated proteins present in the BM were also seen ( Fig. 2a,b ). No changes in E-cadherin staining around the periphery of epithelial cells were observed ( Fig. 2 ), so we therefore used E-cadherin levels as an internal control to quantify changes in the intensity of BM proteins. Reductions in laminin, collagen IV and PNA staining within the BM of Galnt1 −/− SMGs (expressed as a ratio with E-cadherin) were calculated and are shown in Fig. 2b–d . Interestingly, no changes in α6 integrin present along the basal region of the epithelial cells were observed between wild-type and Galnt1 −/− SMGs ( Supplementary Fig. S4 ), suggesting that the effects of Galnt1 loss are specific to these secreted BM proteins. Additionally, no significant differences in laminin or collagen IV gene expression were detected among Galnt1 +/+ , Galnt1 +/− and Galnt1 −/− SMGs ( Fig. 2e ), suggesting that the specific reduction in laminin and collagen in the BM is not due to a reduction in gene expression, but may be due to a defect in secretion. 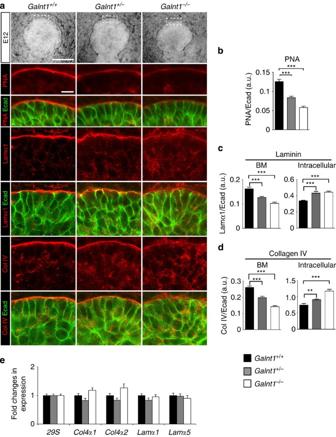Figure 2: Loss ofGalnt1causes reduction in ECM proteins and O-glycans in the BM of E12 SMGs. (a) Phase-contrast images of E12 SMGs (top row) highlight the region (white dashed box) of high-magnification views in the single section confocal images shown below. Immunofluorescence analysis of wild type (Galnt1+/+),Galnt1heterozygotes (Galnt1+/−) andGalnt1-deficient (Galnt1−/−) E12 SMGs revealed a specific decrease in laminin α1 (Lamα1, red), collagen IV (Col IV, red) and O-glycans (detected by the peanut agglutinin lectin, PNA, red) in the BM ofGalnt1−/−SMGs. Additionally, intracellular accumulation of laminin α1 and collagen IV in epithelial cells was observed. No changes in E-cadherin (Ecad, green) were seen inGalnt1−/−SMGs. (b) PNA-staining intensity along the BM region for each genotype (expressed as a ratio relative to total levels of E-cadherin) was graphed. Staining intensities of Lamα1 (c) and Col IV (d) along the BM and within the epithelial cells were graphed. Five SMGs of each genotype from four independent crosses were examined. (e) Expression of major BM genes is unchanged inGalnt1-deficient SMGs. Expression was normalized to29S. Scale bar, 100 μm for Phase-contrast images and 10 μm for confocal images. Student'st-test was used to calculateP-values. **P<0.01, ***P<0.001. Figure 2: Loss of Galnt1 causes reduction in ECM proteins and O-glycans in the BM of E12 SMGs. ( a ) Phase-contrast images of E12 SMGs (top row) highlight the region (white dashed box) of high-magnification views in the single section confocal images shown below. Immunofluorescence analysis of wild type ( Galnt1 +/+ ), Galnt1 heterozygotes ( Galnt1 +/− ) and Galnt1- deficient ( Galnt1 −/− ) E12 SMGs revealed a specific decrease in laminin α1 (Lamα1, red), collagen IV (Col IV, red) and O-glycans (detected by the peanut agglutinin lectin, PNA, red) in the BM of Galnt1 −/− SMGs. Additionally, intracellular accumulation of laminin α1 and collagen IV in epithelial cells was observed. No changes in E-cadherin (Ecad, green) were seen in Galnt1 −/− SMGs. ( b ) PNA-staining intensity along the BM region for each genotype (expressed as a ratio relative to total levels of E-cadherin) was graphed. Staining intensities of Lamα1 ( c ) and Col IV ( d ) along the BM and within the epithelial cells were graphed. Five SMGs of each genotype from four independent crosses were examined. ( e ) Expression of major BM genes is unchanged in Galnt1- deficient SMGs. Expression was normalized to 29S . Scale bar, 100 μm for Phase-contrast images and 10 μm for confocal images. Student's t -test was used to calculate P -values. ** P <0.01, *** P <0.001. Full size image Loss of Galnt1 reduces BM secretion and induces ER stress Further examination of E12 SMGs revealed an increase in intracellular staining for both laminin and collagen IV within the epithelial cells of Galnt1 −/− and Galnt1 +/− relative to wild type littermate controls ( Fig. 2c,d ). These results suggest that the loss of Galnt1 affects secretion of BM components. To further explore this possibility, we examined secretory apparatus components within the SMG epithelial cells. Significant increases in the ER proteins Sec23 and calnexin were measured in the epithelial cells of Galnt1 −/− and Galnt1 +/− SMGs ( Fig. 3a–c ). Additionally, intracellular staining of laminin and collagen IV showed partial co-localization with the ER in cells of Galnt1 −/− and Galnt1 +/− SMGs ( Fig. 3a ), suggesting altered transport of these proteins through the secretory apparatus. As ER expansion and increases in calnexin are hallmarks of ER stress, we next examined whether ER stress and the unfolded protein response (UPR) were induced in Galnt1 −/− SMGs [38] , [39] , [40] , [41] , [42] , [43] . ER stress-dependent splicing of Xbp1 was seen in Galnt1 −/− and Galnt1 +/− SMGs, but not in Galnt1 +/+ littermate controls ( Fig. 3d ). Additionally, ER stress-dependent translation of ATF4 and proteolytic cleavage of ATF6 were also observed in Galnt1 −/− SMGs, further indicating the induction of ER stress and the UPR ( Fig. 3e ). Furthermore, significant increases in the expression of the ER stress genes Calnexin (Canx) and Edem1 , which are involved in protein folding, processing and degradation, were also observed in Galnt1- deficient SMGs relative to wild type ( Fig. 3f ). However, expression of Chop , an ER stress gene involved in the induction of apoptosis, was unaffected in Galnt1- deficient SMGs. Interestingly, these effects are distinct from those observed upon disruption of N-linked glycosylation by treatment with the inhibitor tunicamycin. Loss of N-glycosylation not only affected BM components and inhibited SMG growth, but also disrupted E-cadherin and α6 integrin localization; increased Chop, Canx and Edem1 expression; and induced apoptosis ( Supplementary Fig. S5a–f ). Taken together, our results indicate that loss of Galnt1 disrupts the specific secretion of BM proteins and induces certain aspects of the ER stress response. 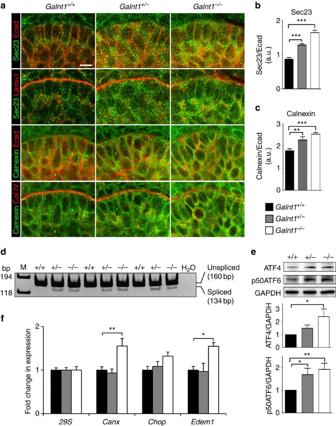Figure 3: Loss ofGalnt1affects secretion of BM proteins and induces ER stress in E12 SMGs. (a) Immunofluorescence analysis ofGalnt1+/+,Galnt1+/−andGalnt1−/−E12 SMGs. SMGs were stained for the ER marker Sec23 (green) and laminin α1 (Lamα1, red) or the ER marker calnexin (green) and collagen IV (Col IV, red) revealed partial co-localization of these BM proteins with the ER inGalnt1−/−SMGs. SMGs were also co-stained with E-cadherin (Ecad, red). Graphs of the ratios of Sec23/Ecad (b) and calnexin/Ecad (c) show an increase in staining for these ER markers inGalnt1−/−epithelial cells. (d) ER stress-dependent splicing of Xbp1 is detected inGalnt1+/−andGalnt1−/−E12 SMGs by PCR. Reaction products in each lane are from cDNA prepared from a pair of E12 SMGs of the genotype denoted above each lane. M=size markers. H2O=control reaction without cDNA added. Negative images of ethidium bromide-stained gels are shown. (e) ER stress-dependent increases in ATF4 protein and the 50kDa cleaved form of ATF6 (p50ATF6) were seen inGalnt1−/−E12 SMGs relative toGalnt1+/+andGalnt1+/−littermate controls. Levels of ATF4 and p50ATF6 were normalized to GAPDH and ratios were graphed. Ratios of AFT4/GAPDH and p50ATF6/GAPDH inGalnt1+/+SMGs were set to 1. Graphs represent the average of five independent experiments for each genotype. (f) Increases in the expression of specific ER stress genes inGalnt1−/−E12 SMGs relative toGalnt1+/+andGalnt1+/−littermate controls. Gene expression levels (from five SMGs of each genotype from three crosses) were determined by qPCR. Expression was normalized to29S. Scale bar, 10 μm. Student'st-test was used to calculateP-values. *P<0.05; **P<0.01; ***P<0.001. Figure 3: Loss of Galnt1 affects secretion of BM proteins and induces ER stress in E12 SMGs. ( a ) Immunofluorescence analysis of Galnt1 +/+ , Galnt1 +/− and Galnt1 −/− E12 SMGs. SMGs were stained for the ER marker Sec23 (green) and laminin α1 (Lamα1, red) or the ER marker calnexin (green) and collagen IV (Col IV, red) revealed partial co-localization of these BM proteins with the ER in Galnt1 −/− SMGs. SMGs were also co-stained with E-cadherin (Ecad, red). Graphs of the ratios of Sec23/Ecad ( b ) and calnexin/Ecad ( c ) show an increase in staining for these ER markers in Galnt1 −/− epithelial cells. ( d ) ER stress-dependent splicing of Xbp1 is detected in Galnt1 +/− and Galnt1 −/− E12 SMGs by PCR. Reaction products in each lane are from cDNA prepared from a pair of E12 SMGs of the genotype denoted above each lane. M=size markers. H 2 O=control reaction without cDNA added. Negative images of ethidium bromide-stained gels are shown. ( e ) ER stress-dependent increases in ATF4 protein and the 50kDa cleaved form of ATF6 (p50ATF6) were seen in Galnt1 −/− E12 SMGs relative to Galnt1 +/+ and Galnt1 +/− littermate controls. Levels of ATF4 and p50ATF6 were normalized to GAPDH and ratios were graphed. Ratios of AFT4/GAPDH and p50ATF6/GAPDH in Galnt1 +/+ SMGs were set to 1. Graphs represent the average of five independent experiments for each genotype. ( f ) Increases in the expression of specific ER stress genes in Galnt1 −/− E12 SMGs relative to Galnt1 +/+ and Galnt1 +/− littermate controls. Gene expression levels (from five SMGs of each genotype from three crosses) were determined by qPCR. Expression was normalized to 29S . Scale bar, 10 μm. Student's t -test was used to calculate P -values. * P <0.05; ** P <0.01; *** P <0.001. Full size image Loss of Galnt1 reduces FGF-mediated cell proliferation To identify the mechanism by which loss of Galnt1 affects SMG growth, we examined cell proliferation in E12 SMGs by EdU incorporation ( Fig. 4 ). A significant reduction in epithelial cell proliferation in Galnt1 −/− SMGs was observed relative to heterozygotes and wild-type SMGs ( Fig. 4a,b ). These results indicate that the decreased growth of Galnt1 −/− SMGs is due to a reduction in cell proliferation. 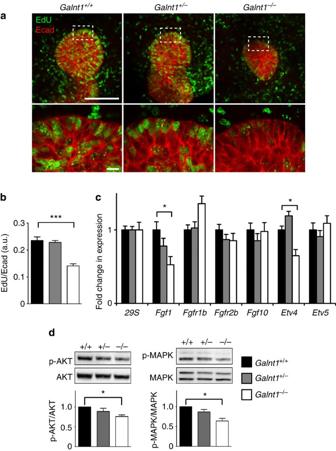Figure 4: Loss ofGalnt1causes reduced cell proliferation and FGF signalling. (a) EdU labelling (green) ofGalnt1+/+,Galnt1+/−andGalnt1−/−E12 SMGs showed decreased epithelial cell proliferation inGalnt1−/−SMGs. Glands were also co-stained with E-cadherin (Ecad, red). The white dash boxes in low-magnification images indicate the location of the high-magnification views below. Scale bars, 100 μm for low magnification and 10 μm for high magnification. (b) Average ratios of EdU/E-cadherin for each genotype are shown. Four SMGs of each genotype from three independent crosses were examined. (c)Fgf1andEtv4expression were specifically decreased inGalnt1−/−E12 SMGs as determined by qPCR. Expression was normalized to29S. (d) Decreased AKT and MAPK phosphorylation was seen inGalnt1−/−E12 SMGs relative toGalnt1+/+andGalnt1+/−littermate controls. Graphs are the average of values obtained from five SMGs of each genotype. Student'st-test was used to calculateP-values. *P<0.05; ***P<0.001. Figure 4: Loss of Galnt1 causes reduced cell proliferation and FGF signalling. ( a ) EdU labelling (green) of Galnt1 +/+ , Galnt1 +/− and Galnt1 −/− E12 SMGs showed decreased epithelial cell proliferation in Galnt1 −/− SMGs. Glands were also co-stained with E-cadherin (Ecad, red). The white dash boxes in low-magnification images indicate the location of the high-magnification views below. Scale bars, 100 μm for low magnification and 10 μm for high magnification. ( b ) Average ratios of EdU/E-cadherin for each genotype are shown. Four SMGs of each genotype from three independent crosses were examined. ( c ) Fgf1 and Etv4 expression were specifically decreased in Galnt1 −/− E12 SMGs as determined by qPCR. Expression was normalized to 29S . ( d ) Decreased AKT and MAPK phosphorylation was seen in Galnt1 −/− E12 SMGs relative to Galnt1 +/+ and Galnt1 +/− littermate controls. Graphs are the average of values obtained from five SMGs of each genotype. Student's t -test was used to calculate P -values. * P <0.05; *** P <0.001. Full size image To determine the signalling pathways involved, we examined the expression of genes known to regulate SMG growth [13] , [44] . qPCR revealed a specific decrease in the expression of Fgf1 and a downstream target gene of Fgfr2b signalling, Etv4, in Galnt1 −/− SMGs relative to wild type and heterozygotes ( Fig. 4c ). Accordingly, in Galnt1- deficient glands, we measured a specific decrease in phosphorylated AKT and MAPK ( Fig. 4d ), two kinases involved in FGF-mediated cell proliferation. Taken together, our data suggest that the loss of Galnt1 affects BM secretion, which influences epithelial FGF-mediated signalling and cell proliferation during SMG development. Exogenous laminin-111 rescues Fgf1 expression and SMG growth To demonstrate that the altered BM in Galnt1- deficient glands is responsible for the reduced growth and FGF signalling observed, we supplemented Galnt1- deficient glands with the major component of the embryonic BM (laminin-111) ( Fig. 5 and Supplementary Fig. S6 ). The addition of laminin-111 to Galnt1- deficient SMGs restored Fgf1 and Etv4 expression as well as SMG growth (as assessed by both bud number and quantification of total epithelial area) ( Fig. 5a–d ). In contrast, laminin-111 had no effect on SMG growth defects resulting from the loss of N-glycosylation ( Supplementary Fig. S5a ). It was previously shown that laminin mediates FGF signalling through β1 integrin in the SMG [12] . We therefore examined whether the laminin rescue of Fgf1 and Etv4 expression was dependent on integrin function by using a β1 integrin function-blocking antibody in the rescue experiments. As shown in Fig. 5d , the β1 integrin function-blocking antibody abrogated laminin-111 rescue of Fgf1 and Etv4 expression and SMG growth. Taken together, our studies demonstrate that Galnt1 influences SMG growth by modulating BM secretion, thereby affecting integrin signalling, AKT/MAPK phosphorylation and FGF signalling. 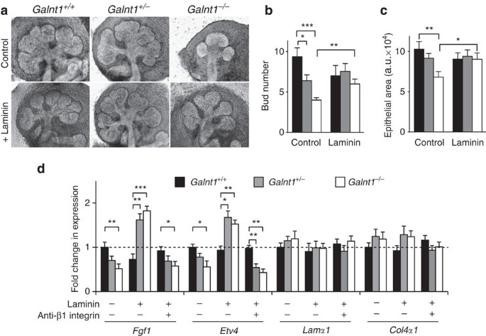Figure 5: Exogenous BM components rescueGalnt1−/−phenotype in a β1 integrin-dependent manner. (a)Galnt1+/+(n=11),Galnt1+/−(n=20) andGalnt1−/−(n=9) E12 SMGs were untreated (Control) or treated with 80 μg ml−1laminin-111 (+ Laminin) for 48 h. The average bud number (b) and epithelial area (c) present after culturing E12 SMGs for 48 h in the presence or absence of laminin revealed that growth was restored inGalnt1−/−SMGs. (d) Laminin addition toGalnt1-deficient SMGs rescuedFgf1andEtv4expression, as determined by qPCR. However, laminin rescue ofFgf1andEtv4expression inGalnt1−/−SMGs is abrogated in the presence of β1 integrin function blocking antibody, as determined by qPCR. Student'st-test was used to calculateP-values. *P<0.05; **P<0.01; ***P<0.001. Figure 5: Exogenous BM components rescue Galnt1 −/− phenotype in a β1 integrin-dependent manner. ( a ) Galnt1 +/+ ( n =11), Galnt1 +/− ( n =20) and Galnt1 −/− ( n =9) E12 SMGs were untreated (Control) or treated with 80 μg ml −1 laminin-111 (+ Laminin) for 48 h. The average bud number ( b ) and epithelial area ( c ) present after culturing E12 SMGs for 48 h in the presence or absence of laminin revealed that growth was restored in Galnt1 −/− SMGs. ( d ) Laminin addition to Galnt1- deficient SMGs rescued Fgf1 and Etv4 expression, as determined by qPCR. However, laminin rescue of Fgf1 and Etv4 expression in Galnt1 −/− SMGs is abrogated in the presence of β1 integrin function blocking antibody, as determined by qPCR. Student's t -test was used to calculate P -values. * P <0.05; ** P <0.01; *** P <0.001. Full size image Here we demonstrate for the first time that loss of an O-glycosyltransferase causes pronounced effects on organogenesis and cell proliferation by altering the secretion of BM components. Our study provides mechanistic insight into how this conserved protein modification can impact developmental events by influencing the formation and composition of this highly specialized cellular microenvironment. The BM contains abundant matrix components, enzymes, proteases and growth factors that act in concert to ensure the proper growth and morphogenesis of the SMG during embryogenesis [7] , [9] , [11] , [12] , [13] , [44] . Previous work has demonstrated that components of the BM as well as the enzymes that modify them are responsible for regulating SMG growth by influencing diverse signalling pathways [7] , [9] , [11] , [12] . In particular, laminin is known to signal through β1 integrins to specifically upregulate Fgf1 , Fgfr1b and Fgfr2b , thereby influencing FGF signalling [12] , [44] . Here we show that the loss of an enzyme responsible for the initiation of O-glycosylation causes intracellular accumulation of laminin and collagen IV, concomitant with a reduction of each in the BM. Specific decreases in Fgf1 expression, AKT and MAPK activation, and SMG growth were also seen in Galnt1 −/− SMGs. Interestingly, addition of exogenous laminin rescued FGF signalling and growth of Galnt1 −/− SMGs in a β1 integrin-dependent manner. Therefore, we propose that the reduction of laminin in the BM of Galnt1- deficient SMGs results in decreased β1 integrin signalling, with subsequent effects on Fgf1 expression, FGF signalling and SMG growth ( Fig. 6 ). This work provides the first example of the loss of an O-glycosyltransferase modulating cell signalling events by influencing the composition of the BM. 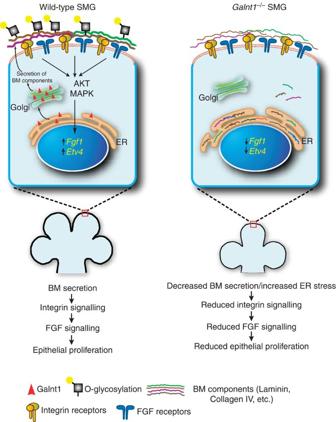Figure 6: Working model showing howGalnt1influences BM composition andFgf1-mediated SMG proliferation. Loss ofGalnt1results in reduced secretion of BM components, causing induction of the ER stress response. Altered BM composition inGalnt1−/−SMGs causes reduced signalling by laminin through β1 integrin receptors, resulting in decreasedFgf1andEtv4expression, reduced AKT/MAPK phosphorylation and reduced epithelial cell proliferation. Figure 6: Working model showing how Galnt1 influences BM composition and Fgf1 -mediated SMG proliferation. Loss of Galnt1 results in reduced secretion of BM components, causing induction of the ER stress response. Altered BM composition in Galnt1 −/− SMGs causes reduced signalling by laminin through β1 integrin receptors, resulting in decreased Fgf1 and Etv4 expression, reduced AKT/MAPK phosphorylation and reduced epithelial cell proliferation. Full size image The specific mechanisms by which Galnt1 affects the composition of the BM are currently under investigation. Previous work in Drosophila demonstrated that the catalytic activity of one family member was essential to mediate proper cell adhesion events by glycosylating a BM protein [45] , [46] . Here the glycosyltransferase encoded by Galnt1 (ppGalNAcT-1) may also directly glycosylate BM proteins, influencing their folding, stability or trafficking through the secretory apparatus. Recent mass spectroscopy studies have demonstrated that many BM proteins, including dystroglycan, agrin and nidogen, are O-glycosylated in mammalian cells [47] . And, while laminin is known to be N-glycosylated, recent studies in both mammalian and Drosophila cells have demonstrated that it is O-glycosylated as well [47] , [48] . Additionally, ppGalNAcT-1-mediated glycosylation of components of the secretory apparatus may also influence the proper trafficking and secretion of BM proteins as well as modulate the ER stress response. Recent work has demonstrated that Golgi and ER proteins known to be involved in secretion, secretory apparatus structure and ER stress are O-glycosylated, including calnexin, HSPA5, LMAN1 and MIA3 (ref. 47 ). Therefore, the direct targets of ppGalNAcT-1 that are responsible for mediating the biological effects observed may be numerous and diverse. However, the secretion changes observed in Galnt1 −/− SMGs affected BM proteins and not others, such as E-cadherin or α6 integrin. This is in contrast to the effects seen on loss of N-glycosylation. Therefore, whereas N-glycosylation has roles in global protein processing and transport, our results suggest a more specific role for Galnt1 in the polarized secretion of certain BM components. Future studies will be focussed on assessing which proteins are specifically glycosylated by ppGalNAcT-1 and how glycosylation influences their functions to mediate the developmental effects observed. This study provides the first demonstration that the loss of a member of the Galnt family can induce ER stress. Although the role of N-glycosylation in protein processing, transport and quality control is well established [22] , [23] , a role for O-linked glycosylation in these processes has not been described. However, recent studies have begun to elucidate a role for Golgi-resident enzymes in proteostasis and the ER stress response. Short interfering RNA-mediated knockdown of Golgi nucleotide sugar transporters (which provide sugar substrates for the glycosylation of macromolecules within the Golgi apparatus) decreased protein secretion and induced the ER stress response, illustrating a connection between the UPR and Golgi-based modifications [49] . Additionally, a key player (ERManI) in the protein quality control system that targets proteins for ER-associated degradation has recently been identified as a Golgi-resident protein (and not an ER-resident protein, as previously thought), providing evidence for the role of the Golgi apparatus in sensing and tagging proteins destined to be degraded via ER-associated degradation [50] . And finally, proteins involved in the ER stress response itself have recently been shown to be O-glycosylated, suggesting a role for this modification in their function [47] . The data presented here demonstrate that the loss of Galnt1 induces the ER stress response and specific components responsible for increased protein folding and degradation, to reduce protein load in the secretory apparatus [38] , [39] , [40] . Interestingly, loss of Galnt1 did not induce the apoptotic branch of the ER stress pathway, suggesting roles for O-glycosylation distinct from those of N-glycosylation. Altogether, these results highlight a dynamic interplay between the ER and the Golgi apparatus (and the enzymes that lie therein) in the regulation of protein processing, transport and quality control. Our studies indicate a crucial role for Galnt1 at early stages of SMG development, when Galnt1 is the most abundantly expressed isoform. Interestingly, the reduction in growth and epithelial proliferation in Galnt1 −/− SMGs at early stages of development has a lasting impact on SMG size, as Galnt1 −/− SMGs remain significantly smaller than wild type at later stages of development and into adulthood ( Supplementary Fig. S3 ). Whether reduced size affects the secretory capacity of the adult SMG is currently under investigation. Additionally, our results also provide evidence that Galnt heterozygosity may have biological consequences under certain circumstances. Although Galnt1 +/− SMGs did not show overt growth defects when analysed directly from the animal, they did display reduced growth when cultured ex vivo , suggesting that the loss of one copy of Galnt1 can influence SMG growth under certain conditions. We hypothesize that Galnt1 heterozygotes may represent a sensitized background, as evidenced by slight but significant changes in laminin and collagen levels present at the BM of Galnt1 +/− SMGs, as well as by changes related to an ER stress response. Thus, although these changes may not affect gland growth in vivo , they may influence SMG growth ex vivo under conditions that do not completely mimic the normal developmental environment. These results provide insight into how the loss of one copy of a Galnt could contribute to disease susceptibility or predisposition by altering the cellular environment slightly, so as to make a cell or tissue more vulnerable/receptive to other genetic or environmental influences. Such a model may explain the heterozygosity of GALNT12 seen in some colon cancer samples from a study demonstrating an association between the development of colon cancer and inactivating mutations in GALNT12 (ref. 30 ). In summary, this study reveals a novel role for one member of the conserved Galnt glycosyltransferase family in BM formation and FGF signalling during mammalian organogenesis. This work provides mechanistic insight into how O-glycosylation influences cell signalling and proliferation during development by regulating BM secretion and the ER stress response. As new genetic linkages are found between Galnt s and various human diseases [51] , the role these enzymes have in the formation of the ECM and regulation of the proteostasis network needs to be considered. Animal breeding The Galnt1 (previously designated ppGalNAcT-1)-deficient mice were the kind gift of Dr Jamey Marth [37] . Galnt1- deficient mice were backcrossed into the C57BL/6NHsd inbred mouse background for at least six generations before analysis [37] . Heterozygous Galnt1 animals ( Galnt1 +/− ) were crossed to generate embryos of the genotypes denoted (ASP protocol #08-498). Embryos were genotyped by PCR according to standard procedures [37] . Wild-type ( Galnt1 +/+ ), heterozygous ( Galnt1 +/− ) and homozygous Galnt1- deficient ( Galnt1 −/− ) siblings were compared in all experiments. Semi-quantitative RT–PCR DNase-free RNA was prepared using an RNAqueous-Micro kit (Ambion) and reverse-transcribed to make complementary DNA (Bio-Rad). Primers for Galnt and ER stress genes were designed using Beacon Designer software (Premier Biosoft) and are shown in Supplementary Tables S1 and S2 . Other primers used were previously published and are available on request [11] , [12] . qPCR was performed for 40 cycles (95 °C for 10 s and 62 °C for 30 s) using SYBR-green PCR Master Mix, 1 ng of each cDNA sample and a My IQ real-time PCR thermocycler or CFX96 Real-Time system (Bio-Rad). Gene expression was normalized to the housekeeping gene 29S . Reactions were run in triplicate, and each experiment was repeated three times. PCR to detect splicing of Xbp1 mRNA Xbp1 PCR was performed using primers shown in Supplementary Table S2 . Briefly, PCRs were performed for 35 cycles (94 °C for 30 s, 61 °C for 30 s and 72 °C for 90 s) in a Veriti ™ thermal cycler (Applied Biosystems), using 10 ng of each cDNA sample. The PCR products were identified using a 4–12% acrylamide gel. Negative images of ethidium bromide-stained gels are shown. Ex vivo SMG organ culture SMGs from different stages were dissected and cultured on Nuclepore filters (VWR), as described [13] . Briefly, the filters were floated on 200 μl of DMEM-F12 in 50-mm glass-bottom microwell dishes (MatTek, MA, USA). The culture medium contained 100 U ml −1 penicillin, 100 μg ml −1 streptomycin, 150 μg ml −1 vitamin C and 50 μg ml −1 transferrin. SMGs were cultured at 37 °C in a humidified 5% CO 2 incubator, and photographed at different time points. The epithelial buds were counted and E12 bud size was measured using ImageJ (NIH) software. Experiments were repeated at least three times. Whole-mount immunofluorescence SMGs were fixed with 4% PFA/PBS for 20 min at room temperature or with methanol/acetone (1:1) for 10 min at −20 °C, and then blocked with 10% donkey serum, 1% BSA and M.O.M. blocking reagent (Vector Laboratories). Primary antibodies were diluted with M.O.M. protein reagent in PBS-0.1% Tween 20 and incubated at 4 °C overnight. The following antibodies were used: Collagen IV (Ab769, Milipore; 1:200); E-cadherin (610182, BD Biosciences; 1:200); Laminin α1 (a gift from Dr Takako Sasaki; 1:100) [52] ; Sec23 (E-19 sc-12107, Santa Cruz; 1:100); Calnexin (NB100-1965, Novus Biologicals; 1:100) and α6 integrin (GoH3, 555734, BD Biosciences; 1:100). After washing, SMGs were incubated with Cy3- and Cy5-conjugated secondary Fab fragment antibodies (Jackson Laboratories) and FITC-conjugated PNA (FL-1071, Vector Laboratories; 1:400). Stained SMGs were mounted and visualized on a Zeiss LSM 510 confocal microscope. Representative single section confocal images are shown in each figure. Images were analysed by NIH ImageJ software and assembled in Photoshop. Fluorescence signal quantification Fluorescent intensity of confocal images was measured using NIH ImageJ software. Briefly, 6 single section confocal images separated by 0.5 μm intervals were obtained for each SMG analysed. Three regions within each single section were used to quantify fluorescent signal intensity and these values were averaged to obtain a value for each marker for a particular SMG. The regions chosen for analysis centred on the BM (for PNA, laminin α1 and collagen IV) (each region was ~70 μm×10 μm in dimension), the epithelial region below the BM (for laminin α1 and collagen IV) (each region was ~70 μm×40 μm) or the epithelial region including the BM (for E-cadherin, α6 integrin, Sec23, Calnexin and EdU) (each region was ~70 μm×50 μm). At least 3 SMGs of each genotype were analysed. Western blotting and analysis Staged SMGs were lysed in RIPA buffer. Paired SMGs from Galnt1 +/+ , Galnt1 +/− and Galnt1 −/− littermates were analysed by SDS–PAGE under denaturing conditions and transferred to nitrocellulose membranes. For AKT/MAPK westerns, membranes were blocked with 5% BSA-TBST and probed with phospho- and total-AKT and MAPK (Erk1/2) antibodies (#9271, #9272, #4376, #9102, Cell Signaling Technology; 1:1000). To assess ER stress proteins by western blot, membranes were blocked with 2% BSA-PBST and probed with ATF4 (WH0000468M1, Sigma-Aldrich; 1:500), ATF6 (PRS3683, Sigma-Aldrich; 1:1000) or GAPDH (sc-25778, Santa Cruz; 1:2000). After washing, membranes were probed with HRP-conjugated anti-mouse IgG (GE Healthcare; 1:5000) or HRP-conjugated anti-rabbit IgG (Cell Signaling; 1:10,000). The HRP signal was detected using a chemiluminescent substrate (Thermo Scientific) and analysed with a Fuji imager. NIH ImageJ was used to measure band intensity, and the ratios of ATF4/GAPDH or ATF6 (50 kDa)/GAPDH were determined for each genotype (setting the ratio for wild-type littermate controls to 1). Detection of cell proliferation SMG epithelial proliferation was detected using the Click-iT 5-ethynl-2′-deoxyuridine (EdU) imaging kit (C10337, Molecular Probes). 5 μM EdU was added to SMG cultures and incubations proceeded for 30 min at 37 °C. SMGs were then fixed in 4% PFA/PBS and permeabilized with 0.1% Triton X-100. Click-iT detection was performed using Alexa Fluor 488 azide. EdU detection is compatible with subsequent antibody and nuclear staining. Laminin rescue experiments E12 SMGs from each animal were separated and cultured, either with or without 80 μg ml −1 exogenously added laminin-111 (3446-005-01, Trevigen, MD, USA). Both treated and untreated SMGs were cultured for 2 days and then epithelial buds were counted and total epithelial area was measured using NIH ImageJ software; RNA was extracted from SMGs to perform qPCR. Preservative-free anti-β1 integrin antibody (Ha2/5) and hamster control IgM (555002, 553957, BD Biosciences) were used for the β1 integrin function-blocking experiments. 50 μg ml −1 anti-β1 integrin antibody or control IgM were added at the beginning of the culture period. 80 μg ml −1 laminin-111 was added after 30 min to both control IgM and β1 integrin antibody-treated SMGs. Cultures were continued for 2 days, after which SMGs were collected for analysis and RNA extraction. Experiments were repeated four times. Statistical analyses Values were plotted as means±standard errors of the mean for each group from three or more experiments. Student's t -test was used to calculate P -values. How to cite this article: Tian, E. et al . O-glycosylation modulates integrin and FGF signalling by influencing the secretion of basement membrane components. Nat. Commun. 3:869 doi: 10.1038/ncomms1874 (2012).